Convergent evolution in locomotory patterns of flying and swimming animals Locomotion is one of the major energetic costs faced by animals and various strategies have evolved to reduce its cost. Birds use interspersed periods of flapping and gliding to reduce the mechanical requirements of level flight while undergoing cyclical changes in flight altitude, known as undulating flight. Here we equipped free-ranging marine vertebrates with accelerometers and demonstrate that gait patterns resembling undulating flight occur in four marine vertebrate species comprising sharks and pinnipeds. Both sharks and pinnipeds display intermittent gliding interspersed with powered locomotion. We suggest, that the convergent use of similar gait patterns by distinct groups of animals points to universal physical and physiological principles that operate beyond taxonomic limits and shape common solutions to increase energetic efficiency. Energetically expensive large-scale migrations performed by many vertebrates provide common selection pressure for efficient locomotion, with potential for the convergence of locomotory strategies by a wide variety of species. Animals use diverse strategies to reduce the energetically expensive cost of locomotion [1] that range from morphological solutions, such as compliant tendons [2] and low drag-coefficients [3] , to behavioural solutions, such as porpoising [4] , selective use of currents and winds [5] or travelling in formation [6] , [7] . One such behavioural strategy, intermittent locomotion, is widely used by both vertebrates and invertebrates to reduce the cost of movement and includes terrestrial, avian and aquatic fauna [8] . Birds in particular use various types of intermittent locomotion to reduce the mechanical power required for horizontal travel [9] , [10] , [11] . Undulating flight is a special form of intermittent locomotion and involves gliding with flexed wings interspersed with active flapping. Potential energy from gravity and altitude is translated into horizontal distance via gliding, which is thought to result in savings of mechanical power compared with continuous level flight [10] , [11] , [12] . Although only described for flying birds and bats, undulating flight could theoretically occur in any fluid environment and reduce the cost of locomotion under the right physical conditions [9] . Recent work using animal-attached tags has revealed that a range of air-breathing marine animals glide during phases of ascents or descents while assisted by buoyancy, which has been attributed to increase dive efficiency through economic transiting from surface to depth [13] , [14] , [15] , [16] . Here we show that intermittent glides of four species of marine vertebrates are analogous to undulating flight as observed in flying animals. A direct comparison of continuous and intermittently swimming seals revealed that during intermittent swimming, less locomotory effort was performed than during continuous swimming at corresponding velocities. 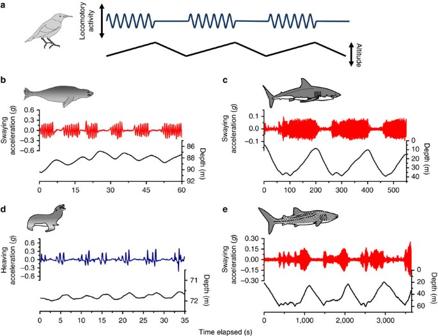Figure 1: Intermittent locomotion in flying and swimming animals. Undulating flight is characterized by altering passive descent gliding and active climbing. (a) Schematic figure of a starling engaged in intermittent flight, adapted from Rayneret al.10Similar patterns are observed in elephant seals (b) and northern fur seals (d) during the bottom phase of dives, white sharks (c) and whale sharks (e) throughout the water-column. Patterns are consistent irrespective of medium (air (a) versus water (b,c,d,e)) and mode of propulsion (pectoral propulsion (a,d), versus caudal propulsion (b,c,e)). Undulating flight in water Animal-attached electronic tags logged acceleration and depth in two species of sharks (whale shark, Rhincodon typus , and white shark, Carcharodon carcharias , Table 1 ) and two species of pinnipeds (northern fur seal, Callorhinus ursinus , and southern elephant seal, Mirounga leonina , Table 1 ). The results reveal that their movement patterns show a high degree of similarity (also see Kawabe et al . [17] ). All four species performed undulating flight, where passive gliding descents are interspersed with ascents characteristic of active propulsion ( Fig. 1 ; Supplementary Movie 1 ). 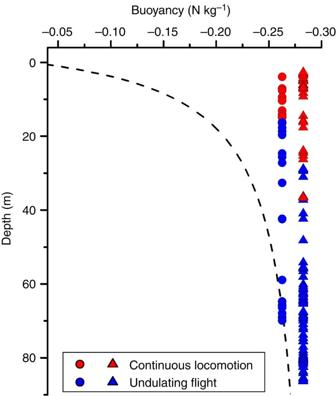Figure 2: Buoyancy and gait patterns in elephant seals. Observed gait patterns in relation to buoyancy conditions experienced by elephant seals. Changes in buoyancy with depth were calculated for an elephant seal based on body composition before migration following the moult (Methods). During the bottom phase of u-shaped dives, elephant seal 1 (triangles) and elephant seal 2 (circles) swam continuously (red) at shallow (<∼15 m) depth and started to adopt undulating flight (blue) at deeper (>∼15 m) depths, where their negative buoyancy was greater. All individuals of the four species exhibited variability in the locomotory power output, the duty factor (the percentage of time spent in active locomotion compared with gliding [18] ), as well as the sink- and climb-rate ( Table 2 ). Elephant seals swam almost exclusively continuously at depths shallower than ∼ 15 m, whereas at deeper depths they adopted intermittent locomotion ( Figs 2 and 3 ). Moreover, duty factor decreased with increasing depth in fur seals (Spearman's ρ =−0.244, P <0.01, n =126), whereas there was no detectable change in whale sharks (Spearman's ρ =0.089, P =0.120, n =308). Table 1 Details of all deployments of acceleration data-loggers on the four species of marine vertebrate. Full size table Figure 1: Intermittent locomotion in flying and swimming animals. Undulating flight is characterized by altering passive descent gliding and active climbing. ( a ) Schematic figure of a starling engaged in intermittent flight, adapted from Rayner et al . [10] Similar patterns are observed in elephant seals ( b ) and northern fur seals ( d ) during the bottom phase of dives, white sharks ( c ) and whale sharks ( e ) throughout the water-column. Patterns are consistent irrespective of medium (air ( a ) versus water ( b , c , d , e )) and mode of propulsion (pectoral propulsion ( a , d ), versus caudal propulsion ( b , c , e )). Full size image Table 2 Characteristics of all undulations (total N =558) for all four species studied. Full size table Figure 2: Buoyancy and gait patterns in elephant seals. Observed gait patterns in relation to buoyancy conditions experienced by elephant seals. Changes in buoyancy with depth were calculated for an elephant seal based on body composition before migration following the moult (Methods). During the bottom phase of u-shaped dives, elephant seal 1 (triangles) and elephant seal 2 (circles) swam continuously (red) at shallow (< ∼ 15 m) depth and started to adopt undulating flight (blue) at deeper (> ∼ 15 m) depths, where their negative buoyancy was greater. 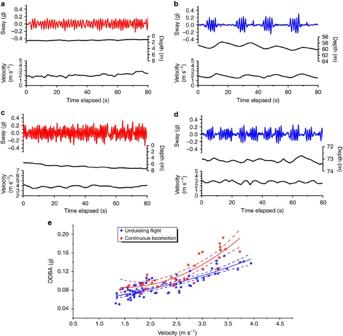Figure 3: Locomotory activity and gait patterns in an elephant seal. Changes in gait associated with the two swimming patterns in a free-swimming southern elephant seal (M. leonina); continuous locomotion (red) at shallow depth with a velocity of 2 m s−1(a) and 3.5 m s−1(c) and undulating flight (purple) at the 2 m s−1(b) and 3 m s−1(d). Power requirements (ascertained via ODBA), (e) increased significantly with swimming-speed in both continuous (y=0.02x2–0.06x–0.13;r2=0.78; F2,31=56.38;P<0.0001 ) and undulating flight corrected for horizontal speed (y=0.004x2+0.007x+0.050;r2=0.74; F2,75=110.10;P<0.0001). 95% confidence intervals are displayed. Full size image Figure 3: Locomotory activity and gait patterns in an elephant seal. Changes in gait associated with the two swimming patterns in a free-swimming southern elephant seal ( M. leonina ); continuous locomotion (red) at shallow depth with a velocity of 2 m s −1 ( a ) and 3.5 m s −1 ( c ) and undulating flight (purple) at the 2 m s −1 ( b ) and 3 m s −1 ( d ). Power requirements (ascertained via ODBA), ( e ) increased significantly with swimming-speed in both continuous ( y =0.02 x 2 –0.06 x –0.13; r 2 =0.78; F 2,31 =56.38; P <0.0001 ) and undulating flight corrected for horizontal speed ( y =0.004 x 2 +0.007 x +0.050; r 2 =0.74; F 2,75 =110.10; P <0.0001). 95% confidence intervals are displayed. Full size image Kinematics and power requirements in continuous and intermittent locomotion The elephant seal carrying speed and acceleration sensors showed significant increases in the duty factor as it increased its swimming speed (cf. Fig. 3 ; y =0.94 x +0.33; r 2 =0.36; F 1,76 =42.43, P <0.0001). Detailed analysis of locomotory effort through the activity metric overall dynamic body acceleration (ODBA) [19] , [20] , which integrates estimated metabolic effort for movement over limb-stroke frequency and amplitude [21] , revealed this elephant seal utilized a smaller range of locomotory power output in 'undulating locomotion' (1st and 3rd quartile of measured ODBA: 0.12 g and 0.14 g , respectively) compared with continuous locomotion (1st and 3rd quartile of measured ODBA: 0.09 g and 0.15 g , respectively). A direct comparison of undulating flight and continuous locomotion at corresponding velocities revealed that the elephant seal engaged in less locomotory power output (as ascertained by ODBA) while swimming intermittently ( Fig. 3 ). Assuming an underlying linear relationship of ODBA and oxygen consumption [19] , [20] , [22] , the elephant seal saved between 13% and 35.6% of activity-related metabolism by utilizing intermittent locomotion at depth greater than ∼ 15 m compared with continuous locomotion at shallower depths ( Fig. 3 ). At routine horizontal travel speeds of <2.5 m s −1 , ODBA of undulating swimming (0.081±0.015 g ) was significantly lower (Mann−Whitney- U test, U (69)=226, Z =−2.881, P <0.01) compared with continuous swimming (0.093±0.010 g ), representing a mean saving of ∼ 13%. Our results show that intermittent locomotion, analogous to undulating flight, is found in a range of marine species, such as sharks and seals ( Fig. 1 ; also see Kawabe et al . [17] ).This high degree of similarity in the movement patterns of the different species is surprising considering their distinct evolutionary history and differing modes of propulsion; fur seals swim by pectoral propulsion, elephant seals use modified hind limbs as flippers and sharks propel themselves using a caudal fin. The intermittent locomotion observed was associated with changes in depth, thus resembling undulating flight described in birds ( Fig. 1 ; Supplementary Movie 1 ). Mechanical models have shown that modest to significant savings of metabolic power can be achieved by undulating flight in both air and water [9] , [10] , [23] . Most aquatic studies have focused on the metabolic savings that are achieved while animals are assisted by buoyancy [13] , [14] , [15] , thus losing potential energy that has to be repaid (but see Davis & Weihs [16] ). Indeed, such studies have focused on locomotory adjustments to changing buoyant forces as pulmonary and fur associated air is compressed with increasing depth, resulting in less stroking and more gliding. In contrast, our study shows that intermittent locomotion is also an effective mode of locomotion when the net change in potential energy is zero, that is, no net change of depth ( Figs 1 and 3 ) and buoyancy remains near constant, as the amplitude of individual undulations is too small to elicit a significant change in the volume of respiratory and fur-associated air. As ODBA has been shown to correlate linearly with oxygen consumption in the exercising marine and terrestrial animals examined thus far [19] , [20] , [22] , our treatise demonstrates that muscular work is more pronounced in continuous locomotion than in intermittent locomotion. The kinematics of undulating flight vary according to travel speed and morphology in birds [11] and we observed a similar relationship in our marine vertebrates ( Table 2 ; Fig. 3 ). Indeed, similar to the elephant seal in this study ( Fig. 3 ), birds performing undulating flight have been shown to increase duty factor with flight speed. It is thought that this modulation of duty factor permits birds to maintain relatively constant wing-beat kinematics resulting in maximum efficiency [11] , although it is still debated whether birds perform undulating flight because of kinematic and muscular constraints, rather than purely to save mechanical work [10] , [11] . It is therefore interesting that the elephant seal was able to satisfy mechanical power requirements for the same range of speeds using continuous and intermittent stroking, suggesting that intermittent locomotion primarily serves energy conservation in this species. However, the resultant saving is presumably a combination of efficiently converting muscular power into thrust, which relies on the interaction of an efficient muscle working stroke, coupled with limb kinematics that maximize the overall economy of converting fuel into forward locomotion. Whereas the kinematics of individual undulations where relatively invariant in the pinnipeds, vertical movement during undulation in sharks displayed larger plasticity ( Table 2 ). This variance was likely due to varying motivation of movement, given that large scale vertical movements serve both the purpose of travel and search in sharks [23] , [24] , which are characterized by different optima [25] . Indeed, the amplitude of individual undulations by sharks occurred over a wide vertical range (2–70 m, Fig. 1 ), whereas amplitudes were far more constrained in the two species of seal ( Table 2 ). Despite the large variability in diving patterns of whale sharks, a recent study was able to show that continuous bounce diving utilized descent and ascent angles, which optimize the horizontal cost of transport [25] , supporting the notion that sharks also move through the water column in order to cover horizontal distance efficiently. These lines of evidence substantiate theoretical evidence of the efficacy of intermittent locomotion for the reduction of the cost of transport. Marine animals are often neutrally buoyant at depth, which yields insights into undulating flight as a gait in air and water. We found no evidence of intermittent locomotion by elephant seals at depths shallower than ∼ 15 m ( Figs 2 and 3 ), probably as a result of animals being near neutral buoyancy ( Fig. 2 ) [26] , whereas at deeper depths seals would swim intermittently, likely due to their increased overall density ( Fig. 2 ). The lack of gas-spaces in sharks results in a fixed body density greater than that of water, irrespective of depth [27] , [28] . Thus, sharks can exhibit larger amplitudes in individual undulations than the two species of pinnipeds ( Table 2 ). In fact, the amplitudes of the undulations in seals were so small that variations in body density are likely to be inconsequential within peaks and troughs of each undulation ( Table 2 and Fig. 2 ), in a manner similar to the fixed negative buoyancy of sharks. However, there were significant differences in the depth at which the two elephant seals started to swim intermittently, likely resulting from differing body density ( Fig. 2 ) [29] . Swimming gaits have been shown to relate to body condition in a number of species, such as baikal seals ( Pusa sibirica ) and weddel seals ( Leptonychotes weddellii ), with seals of higher body density adopting more gliding behaviour during descent [30] , [31] . It is, however, possible that a shift in behavioural mode, rather than buoyancy alone, triggered a change in the gait pattern of the elephant seals. For instance, some species of primate adopt intermittent locomotion to scan the environment, which may enable more efficient prey detection [8] . Against this, our elephant seal was on the outward leg of its migration moving rapidly over the Patagonian Shelf towards the shelf edge using u-shaped dives characteristic of directed travelling, whereas deep dives indicating foraging only occur once off-shelf waters are reached [32] supporting the notion that energy conservation is the prime reason for intermittent locomotion. Our results suggest that effective intermittent locomotion may require potential energy to be translated into horizontal distance and that seals have to exceed a critical body density to undulate effectively. Indeed, whereas duty factor increased systematically with depth in fur seals, which are characterized by appreciable air in their pelage, no such pattern was evident in whale sharks, presumably due to the lack of airspaces in sharks. Sharks, with their depth-independent negative buoyancy, appear to be able to glide continuously throughout the water column, whereas seals appear to be constrained to the depths were they attain negative buoyancy [30] . These results are at odds with 'burst and coast' swimming in small teleost fish, which may occur as a consequence of the profound difference in size between the fish observed thus far, and our study subjects. Indeed, it is possible that the cost of the burst acceleration phase is mass-specific [33] and larger animals may benefit from less deceleration during the coast phase, which may be enhanced by negative buoyancy. In addition, locomotory activity during the active phase shows complete overlap with continuous locomotion, suggesting that undulating flight in large marine vertebrates is aerobic, unlike burst-coast swimming in smaller fish. The advantage of negative buoyancy as shown by our study has profound implications for our understanding of optimal body density in aquatic animals, where historically neutral buoyancy is often considered advantageous. In all likelihood, there is probably no single density that is optimal under all circumstances. Adjustment of density is likely highly adaptive, such that aquatic animals that exploit a prey patch at a given depth will benefit from neutral buoyancy [34] , while travelling animals may benefit from negative buoyancy ( Figs. 2, 3 ). While many of the pelagic fish species have a reduced swim-bladder, there remains fine volume control over the size of the gas bladder. Our findings indicate that intermittent locomotion in marine environments may be a common mode of transport that in all likelihood favours a lowering of aerobic costs due to efficient locomotion. By using animal-attached technologies to study submerged marine vertebrates, we demonstrate that this strategy operates in water across taxonomic clades as well as in air. Indeed, the species studied here all have to complete large-scale migrations between patches of productivity [35] , [36] , [37] , which would make efficient transiting particularly important. Any reduction in the cost of transport is expected to be highly selected for in natural populations and similar constraints are presumed to result in a convergence of morphological or behavioural solutions [38] . Given that animal movement is shaped by universal physical and physiological principles; such as commonalities regarding muscle efficiency [39] and hydrodynamic interactions with the fluid environment [40] , common solutions might be expected to increase energetic efficiency even in differing media [41] . Indeed, sufficient lift-production during glides is the main criterion allowing birds to undulate [11] , [42] , whereas marine animals appear at times to face the opposite problem of not having enough 'effective weight' to undulate. Field protocols We instrumented four species of marine vertebrates from two distinct taxa with data-loggers containing acceleration and depth sensors to record changes in locomotory activity with depth. We attached multisensor data-loggers [42] , very high frequency (VHF) transmitters and platform terminal transmitters (PTTs) to the head of five lactating female southern elephant seals ( M. leonina ) at Peninsula Valdez (42° 44′ S 63° 38′ W), Argentina in October 2008. Animals were equipped before their migration following parturition [32] . Devices were recovered after animals returned from their ∼ 80 days foraging trip. Five data-loggers were deployed on lactating female northern fur seals ( C. ursinus ) on St Paul Island, Alaska (57°6′ N, 170°18′ W), USA during the breeding season of July 2008. Animals were captured and equipped in the rookery and devices recovered after a single foraging trip. Thirteen data-loggers were attached to whale sharks ( R. typus ) at Ningaloo Reef, Western Australia (22°00′S, 113°50′ E) between April and June from 2007–2009 (for full details of the equipment and procedure see Gleiss et al . [43] 43). Three data-loggers were deployed on white sharks ( C. carcharias ) at the Farallon Islands (37°41′ N, 123°00′ W), central California in 2008 and 2009. Data-loggers were hidden in whale blubber obtained from stranding mortalities and freely ingested by sharks attracted to the research vessel. Acceleration data-loggers were attached to a satellite-linked Pop-up archival tag (MK10 Wildlife Computers) via wire-clamps (ClampTite). In addition, more syntactic foam was added to the package to offset the increased specific gravity by the acceleration data-logger. Loggers were recovered after the animal would regurgitate the package and it reported via pop-up satellite tag. By examining the location data provided by the ARGOS system the tag was recovered at sea using ultra high frequency antenna. Device specifications In this study, we employed two basic animal-attached recording systems: a multisensor data-logger [42] and a pop-up satellite archival tag [44] . The multisensor data loggers used are described in detail in Wilson et al . [42] In brief, acceleration and depth are recorded at a fixed frequency, which was determined according to the species in question ( Table 1 ). Acceleration data were calibrated by rotating devices through known angles, so that device output corresponds to g (9.81 ms −2 ). Estimates of locomotory activity were derived through the proxy ODBA [19] , which scales linearly with oxygen consumption in exercising animals [19] , [22] , as a result of the interaction between muscular work and acceleration of the centre of mass [21] . Calibration of the speed sensor Only one of the elephant seals had a long enough data-record to adequately calibrate the on-board speed sensor, which has previously been described by Shepard et al . [45] . This sensor uses a reflective paddle and infrared sensor to measure in water speed, by measuring the amount of infrared reflectance from the paddle, which is a function of distance between the fixed sensor and flexible paddle. To calibrate device output to swimming speed [46] , we calculated the swimming speed for 10-s segments from animal pitch (via the surging acceleration) and vertical velocity (ascertained via pressure sensors) to gain an independent measure of travelling speed. This method is subject to increasingly large error as pitch nears horizontal and we therefore selected regions in the dataset where pitch was greater than 20° from the horizontal. We subsequently regressed calculated speeds with infrared device readings to obtain a predictive relationship, which we applied to the entire dataset. The instrument was only recording data for the portion of the migration where animals were swimming over the shelf, thus resulting in relatively shallow dives (<100 m) and correspondingly shallow pitch angles (mean pitch used to calculate speed was 45±13°), which resulted in larger variance in the calibration compared with other studies where only very steep pitch angles were used (velocity=1 E +50*IR −12.44 , n =51, r 2 =0.71) [46] . Calculation of overall dynamic body acceleration ODBA was calculated following the formulation presented in Wilson et al . [19] ; static acceleration due to gravity was determined using a filter based on adjacent averaging. The size of the filtering window was determined using the method described in Shepard et al . [47] Static acceleration was subsequently subtracted from the raw acceleration to yield dynamic acceleration (acceleration due to motion). This was performed for all three acceleration channels representing the three spatial planes. Absolute values were subsequently added to yield a single proxy for mechanical power output. Mathematically, this can be expresses as: Where a acceleration in x , y or z axis, p is the smoothing window. Data extraction We defined undulating flight as a complete cycle in which the animal intersperses active propulsion with passive gliding, with depth increasing during glides and decreasing during active propulsion. We extracted individual undulations from all species when any flap-glide cycle began and ended at the same depth (we arbitrarily used ±15% offset between ascent and descent depth to qualify for this) in order to minimize error in calculating relative time spent stroking in relation to gliding. We then calculated the total cycle duration of each flap-glide cycle and the time spent gliding and actively stroking to calculate the duty factor the percentage of each movement cycle spent actively stroking [10] . Furthermore, we recorded minimum and maximum depth of each undulation to calculate the amplitude (change in depth over every flap-glide cycle) and the vertical velocity during the descent ('sink-rate') and the ascent ('climb-rate'). In addition, we extracted the mean ODBA for complete undulations as well as during continuous locomotion, in order to compare mean locomotory activity between the two gaits. For the elephant seal, we also manually extracted the mean swim speed for both continuous swimming and undulating flight. To compare the horizontal velocity of undulating flight with that of continuous locomotion, we adjusted the swim speed ( V ) to horizontal velocity ( V Horizontal ), using the absolute pitch angle of ascent and descent (Φ) calculated from the surging acceleration: How to cite this article: Gleiss, A.C. et al . Convergent evolution in locomotory patterns of flying and swimming animals. Nat. Commun. 2:352 doi: 10.1038/ncomms1351 (2011).